Tuning charge–discharge induced unit cell breathing in layer-structured cathode materials for lithium-ion batteries For LiMO 2 (M=Co, Ni, Mn) cathode materials, lattice parameters, a ( b ), contract during charge. Here we report such changes in opposite directions for lithium molybdenum trioxide (Li 2 MoO 3 ). A ‘unit cell breathing’ mechanism is proposed based on crystal and electronic structural changes of transition metal oxides during charge-discharge. Metal–metal bonding is used to explain such ‘abnormal’ behaviour and a generalized hypothesis is developed. The expansion of the metal-metal bond becomes the controlling factor for a ( b ) evolution during charge, in contrast to the shrinking metal-oxygen bond as controlling factor in ‘normal’ materials. The cation mixing caused by migration of molybdenum ions at higher oxidation state provides the benefits of reducing the c expansion range in the early stage of charging and suppressing the structure collapse at high voltage charge. These results may open a new strategy for designing layered cathode materials for high energy density lithium-ion batteries. Since lithium-ion batteries (LIBs) were first commercialized in the early 1990s (ref. 1 ), they have emerged as the most important power sources for portable electronics [2] . However, to expand the applications of the LIBs to electric vehicles, higher energy density and longer cycle life are urgently required. The significant improvements of these two key characters are critically depending on the development of new cathode materials as well as the improvements of the existing ones, which relies on the in-depth fundamental understanding of the structural change mechanisms during charge–discharge cycling of the cathode materials. The widely used commercial cathode materials for LIBs in today’s market are transition metal oxides with layered structure such as LiMO 2 (M=Co, Ni and Mn) [3] , [4] , [5] . The layer-structured LiMO 2 has the theoretical capacities ~270 mAh g −1 ; however, only ~140–150 mAh g −1 reversible capacity can be practically utilized [6] with a cutoff voltage of ~4.2–4.3 V. If the cells could be charged to higher voltages without damaging the structure, higher practical energy density (with high capacity and voltage) would be obtained. Unfortunately, when charge voltage limit is increased above 4.3 V, the reversible capacity in subsequent cycles fades seriously because of the structural degradation caused by high voltage charging [7] , [8] , [9] , [10] . Therefore, redesigning the chemical contents and crystal structures to suppress such structural degradation will open a new approach for developing high energy density cathode materials with long cycle life. This is the main motivation of this work. The layered cathode materials have the hexagonal structure with (R-3m) symmetry. They can be viewed as alternatively stacked close-packed Li layers sandwiched between two O–M–O ‘slabs’ along the c direction [11] . Most of the layer-structured materials have O3-type stacking. During delithiation (charge), Li ions are extracted from the Li layers leading to increased repulsion force between the two neighbouring oxygen layers, causing the increased lattice parameter c of the unit cell. In the meantime, the parameters a and b decrease because of the shrinking M–O bonds in MO 6 octahedral, as a result of contracting ion radius of M with higher oxidation states. During lithiation (discharge), the changes of parameters reverse directions. This type of structural changes is called ‘unit cell breathing’. For LiMn 2 O 4 spinel materials with cubic structure, the unit cell breathing is similar but the lattice parameters contract (during charge) and expand (during discharge) simultaneously in all three directions [12] . When a significant amount of Lis were removed from the layer-structured material during high voltage charging (for example, 50% for LiCoO 2 ), the change of parameter c reversed course from expanding to contracting and can reach values even shorter than the pristine, if charged to voltages close to or higher than 5 V (ref. 8 ). This will cause irreversible structure damage and capacity fading. It is believed that this irreversible damage is caused by the ‘collapse’ of the structure in the c direction because of the almost empty Li layers. If the lattice parameter breathing ranges during cycling can be reduced, the cycle life will be improved. If the structure collapse in the c direction during high voltage charging can be reduced by structural redesign, both the energy density and cycle life can be significantly enhanced. To suppress the collapse in the c direction, we need to get some pillar ions in the empty Li layers to stabilize the structure. To suppress the lattice parameter ‘breathing’ range, we need to find structures and related elements with ‘abnormal’ breathing behaviour other than the Mn-, Co- and Ni-based layer-structured materials (parameter changing in opposite directions). Such materials have been reported in the literature [13] , [14] , [15] , [16] . For example, LiVO 2 shows increased parameters a and b but decreased parameter c during charge [13] , and LiNbO 2 also shows increased parameters a and b , but an unchanged parameter c during delithiation [14] . Kumada et al. [15] investigated the structure changes of lithium molybdenum trioxide (Li 2 MoO 3 ) with disordered α-NaFeO 2 -type layer structure during chemical delithiation up to Li 2− x MoO 3 ( x =0.77). They found that the evolution of lattice parameter change can be divided into two parts: in the region of 0< x <0.51, both parameters a (as well as b ) and c increase with increasing x (delithiation), In the region of 0.51< x <0.71, the parameter a (and b ) continuously increases, while parameter c remains unchanged. Recently, Sathiya et al. [16] reported a new layer-structured cathode material Li 2 Ru 0.75 Sn 0.25 O 3 . It also shows expanding parameters a and b (which we call ‘abnormal’) and contracting parameter c during charge. The reason that we call these behaviours ‘abnormal’ for the lattice parameter changes is based on the fact that they do not follow the ‘normal’ behaviours of Mn-, Co- and Ni-based materials with unit cell volume changes basically synchronized with the changes of metal ion radii. Unfortunately, these ‘abnormal’ lattice parameter changes have not been systematically studied to understand their origin and mechanism. We believe that the in-depth understanding on these abnormal behaviours is very important, since they can be utilized to compensate the lattice parameter changes of the Mn-, Co- and Ni-based ‘normal’ materials to reduce the internal strain and stress during electrochemical cycling, providing new approaches for developing new cathode materials with higher energy density and long cycle life. Here we use Li 2 MoO 3 as a model layered compound with abnormal lattice parameter changes upon electrochemical delithiation to study these interesting phenomena through the point of view of crystal and electronic structural changes. The structure evolution of Li 2 MoO 3 upon charge was studied thoroughly by using synchrotron-based in situ X-ray diffraction (XRD) and X-ray absorption spectroscopy (XAS), as well as spherical-aberration-corrected scanning transmission electron microscopy (STEM). A general relationship hypothesis between the lattice parameter changes and the electronic structure of both ‘normal’ and ‘abnormal’ layer-structured transition metal oxide compounds upon delithiation is proposed. Structure evolution by in situ XRD Li 2 MoO 3 with a disordered α-NaFeO 2 structure has been reported in the literature [17] , [18] . It has a similar layered structure as Li 2 MnO 3 , but with different atom arrangement in the LiM 2 (M=Mn, Mo) plane. In case of Li 2 MnO 3 , Li and Mn ions in the LiMn 2 plane has the ordered distribution (…–Li–Mn–Mn–… in a and b directions) [19] , [20] . In Li 2 MoO 3 , three Mo atoms form a Mo 3 triangle (Mo 3 O 13 cluster), which is distributed randomly in the LiMo 2 plane [18] (the comparison of the structure of LiMn 2 and LiMo 2 planes are shown in Supplementary Fig. 1 ). The in situ XRD patterns of Li 2 MoO 3 upon the first charge are shown in Fig. 1 . The patterns for fully charged and pristine Li 2 MoO 3 are plotted in Fig. 1a,c , respectively. All the peaks can be indexed by a layered structure with the space group R-3m, except for one strong peak at 38.5°, which is from the Al current collector. To demonstrate the phase transition clearly, the contour plots of peak intensity and position for several main peaks as a function of capacity during charge are presented in Fig. 1b . It should be noted that the (003), (107) and (108) peaks mainly reflect the evolution along the c axis, while the (110) and (101) peaks reflect the evolution along the a (and b ) axis. The initial charge curves are shown on the right side in Fig. 1d . In the region of 0< x <0.5, with a voltage slope from 3.0 to 3.6 V, all of these peaks shifted to the lower angles, indicating a solid solution reaction with decreasing d-spacing for Phase I. In the region of 0.5< x <1.0, a new phase (Phase II) started to form and grow at the expense of Phase I. The new phase has the same layered structure as Phase I but larger unit cell with increased lattice parameters in both a ( b ) and c , migrated Mo ions into the original Li layers, as the number of Li ions decreasing (Structure schematics of Phase I and Phase II are shown in Fig. 1 ). The detailed migration of Mo ions into Li layers will be discussed later in the STEM results. A flat voltage plateau can be observed in this region, suggesting a two-phase reaction region. 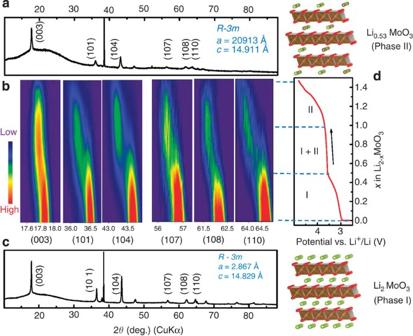Figure 1:In situXRD of Li2MoO3during the first charge. (a) The XRD pattern of the Li2−xMoO3electrode right after charging to 4.8 V. (b) Contour plot of diffraction peak evolution of (003), (101), (104), (107), (108) and (110) during delithiation. (c) The XRD pattern of the Li2MoO3electrode before charge. (d) Charge curve at a current density of 10 mA g−1from open circuit voltage (OCV) to 4.8 V during XRD data collection. When the lithium was further extracted to x >1.0, the original phase disappeared and a continued solid solution reaction of phase II was observed, corresponding to the voltage slope from 3.7 V to the end of charge at 4.8 V. Figure 1: In situ XRD of Li 2 MoO 3 during the first charge. ( a ) The XRD pattern of the Li 2− x MoO 3 electrode right after charging to 4.8 V. ( b ) Contour plot of diffraction peak evolution of (003), (101), (104), (107), (108) and (110) during delithiation. ( c ) The XRD pattern of the Li 2 MoO 3 electrode before charge. ( d ) Charge curve at a current density of 10 mA g −1 from open circuit voltage (OCV) to 4.8 V during XRD data collection. Full size image Each XRD pattern during charge was refined using Le Bail fitting with the R-3m structure. The corresponding lattice parameters obtained are shown in Fig. 2 . From x =0 to 1.0, parameter a of phase I increased from 2.867 to 2.886 Å, and parameter c increased from 14.829 to 14.854 Å. It should be noted that the percentage expansion of parameter c is not as much as that of a . It means that the c / a ratio decreases during charge for Phase I. Such anisotropic change suggests that Li ions are mainly removed from the LiMo 2 layers in this region [16] . All lattice parameters of Phase II are larger than those for Phase I. They also show an increasing trend in the range of 0.5< x <1.47. The three-dimensional (3D) expansion during delithiation for the layered cathodes is quite abnormal. It is well known that parameters a and b for most of LiMO 2 (M=Co, Ni and Mn) materials decrease, while the parameter c increases during delithiation [7] , [8] , [9] , [11] ( Table 1 ). The contracting a and b values for these materials are attributed to the decreasing cation radius of transition metal at higher valence states. The expansion of c is considered to be caused by the increased repulsive force between the MO 2 layers resulting from the reduced number of Li ions in the Li layer. LiMn 2 O 4 spinel with cubic structure shows a contraction in all three dimensions during delithiation [12] . However, if unit cell volume is used to measure the lattice changes, both LiMO 2 (M=Co, Ni and Mn) and LiMn 2 O 4 have decreasing unit cell volume during lithium extraction. It is also true for olivine structured LiFePO 4 (ref. 21 ). It is worthwhile to point out that the c parameter of Li 2 MoO 3 keeps increasing until the end of charge at voltage as high as 4.8 V, indicating a good structure stability in high voltage charging. This is quite different from those widely used LiMO 2 (M=Co, Ni and Mn) systems, which usually show severely decreased parameter c after charging to voltages higher than 4.3 V because of the ‘collapse’ of the structure in the c direction. During the first discharge, the decreasing lattice parameters a and c of Li x MoO 3 changed back to close to the original values (from 2.913 to 2.871 Å for a and 14.911 to 14.831 Å for c , see Supplementary Figs 2 and 3 ). The structure and lattice parameter changes of Li 2 MoO 3 during the second cycle exhibit similar evolution trend as the initial cycle as shown in Supplementary Fig. 4 . 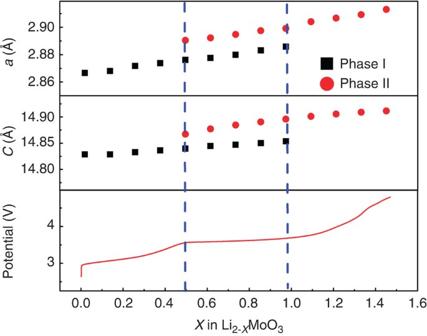Figure 2: Lattice parameter changes of Li2MoO3during the first charge. Lattice parameters of selected XRD patterns were calculated by Le Bail fitting with a R-3m space group. Two phases were identified and marked as Phase I and Phase II. Figure 2: Lattice parameter changes of Li 2 MoO 3 during the first charge. Lattice parameters of selected XRD patterns were calculated by Le Bail fitting with a R-3m space group. Two phases were identified and marked as Phase I and Phase II. Full size image Table 1 Lattice parameter change of layered compounds during delithiation. Full size table For most of the intercalation compounds as cathode materials for lithium batteries, the contraction of the unit cell volume is a ‘normal’ trend during delithiation. It can be generally explained by the shrinking cation radius that resulted from the transition metal oxidation. However, there are several exceptions in the layered Li x MO 2 family ( Table 1 ). LiVO 2 shows a contraction along the c axis and an expansion along the a (and b ) axis during delithiation [13] . The unit cell volume remains approximately the same. Such a contraction in c was explained by the migration of the V ions from the VO 2 layer to the Li layer, which can pull the two adjacent O–V–O slabs closer and lead to decreasing parameter c . LiNbO 2 shows increasing parameters a and b , and an unchanged parameter c upon delithiation [14] , which implies a volume expansion of the unit cell. The unchanged parameter c was considered as the results of the balance between expanded O–Li–O distance and contracted O–Nb–O slab. The increase in the parameters a and b was attributed to the weakening of the Nb–Nb metallic bonding in O–Nb–O slabs. Recently, it was reported that Li 2 Ru 0.75 Sn 0.25 O 3 shows expanded parameter a ( b) and contracted parameter c during charge [16] , while Li 2 Ru 0.5 Mn 0.5 O 3 shows unchanged lattice parameters before 1.2 Li was extracted but contracted parameters a , b and c during further delithiation [22] . In the case of Li 2 MoO 3 we studied here, all the three lattice parameters a , b and c were increased during delithiation. In situ XAS To understand the abnormal structural changes of Li 2 MoO 3 during lithium extraction, in situ XAS at Mo K-edge was applied to monitor the valence state changes of Mo and local structure changes of Li 2 MoO 3 during charge process. 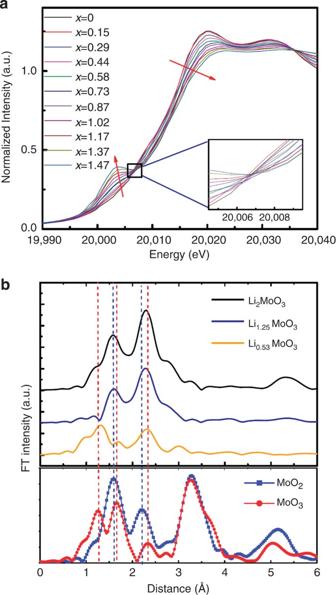Figure 3: XAS spectra of Li2MoO3during the first charge. (a)In situXANES spectra at Mo K-edge during charging to 4.8 V. (b)Ex situFT-EXAFS spectra of Li2−xMoO3at pristine (x=0), half charged (x=0.75) and fully charged (x=1.47) states. The lower panel shows the FT-EXAFS spectra of MoO2anda-MoO3references. Figure 3a shows the X-ray absorption near edge structure (XANES) spectra of the Mo K-edge during charge. A continuous increase in the pre-edge intensity indicates the increased distortion of Mo-O 6 octahedra. Such a pre-edge structure is originated from a quadruple excitation, which is forbidden under perfect octahedral symmetry. This Mo-O 6 octahedra distortion-caused pre-edge structure is the typical feature of a -MoO 3 with Mo 6+ oxidation state. The observation of the increased pre-edge structure and the shifting of the white line to higher energy positions suggests that Mo ions are oxidized to higher than Mo 4+ states upon charging. Compared with the Mo K-edge XANES data of the MoO 2 and a -MoO 3 references ( Supplementary Fig. 5 ), it can be estimated that the Mo ions were oxidized from Mo 4+ to a higher oxidation state between Mo 5+ and Mo 6+ . As shown in the enlarged inset of Fig. 3a , we can see that the intersection is not exactly an ‘isosbestic point’. It should be due to the fact that the charge process of Li 2 MoO 3 is not a simple two-phase reaction, but also includes two solid-solution regions. This is confirmed by the in situ XRD data. Figure 3: XAS spectra of Li 2 MoO 3 during the first charge. ( a ) In situ XANES spectra at Mo K-edge during charging to 4.8 V. ( b ) Ex situ FT-EXAFS spectra of Li 2− x MoO 3 at pristine ( x =0), half charged ( x =0.75) and fully charged ( x =1.47) states. The lower panel shows the FT-EXAFS spectra of MoO 2 and a -MoO 3 references. Full size image Figure 3b shows the magnitude plot of Fourier-transformed extended X-ray absorption fine structure (FT-EXAFS) spectra for Mo K-edge ( k 3 -weighted in k -space) of pristine ( x =0), half charged ( x =0.75) and fully charged ( x =1.47) Li 2− x MoO 3 . The FT magnitudes of MoO 2 and a -MoO 3 are also plotted in the bottom panels as references. For the pristine Li 2 MoO 3 , two dominant peaks can be observed. The peak at ~1.6 Å is assigned to the single scattering path from Mo to the closest oxygen atoms (Mo-O bond in Mo-O 6 octahedra), while the peak at R =~2.3 Å is attributed to the Mo–Mo bonding between two edge-sharing Mo-O 6 octahedra. It should be noted that the FT-EXAFS spectra were not phase-corrected. Therefore, the actual bond lengths are ~0.3–0.5 Å longer. When the sample was charged to Li 1.25 MoO 3 , both of these two main peaks shifted to slightly larger distance and became broader. After further delithiation to Li 0.53 MoO 3 , the spectrum changed completely. Comparing with the FT-EXAFS spectra of MoO 2 and a -MoO 3 references, the peaks at 1.3, 1.7 and 2.1 Å (corresponding to the actual bond length of ~1.6, 2.0 and 2.4 Å after phase correction) for Li 0.53 MoO 3 have the similar bond length values as those for a -MoO 3 , but with different intensity ratios. In the crystal structure of a -MoO 3 , a series of bilayers that are oriented perpendicular to the y axis consists of two sublayers of highly distorted Mo-O 6 octahedra as reported in the literature [23] . There are mainly three different Mo-O bond lengths around 1.7, 2.0 and 2.3 Å in the distorted Mo-O 6 . From the EXAFS spectra, it can be concluded that the Mo-O 6 octahedra in Li 0.53 MoO 3 are severely distorted, just like those in a -MoO 3 . The least-square fitting results of the FT-EXAFS spectra for the pristine Li 2 MoO 3 and charged Li 0.53 MoO 3 are shown in Supplementary Fig. 6 . The phase-corrected structural parameters obtained are listed in Supplementary Table 1 , which shows that the original Mo-O bonds in pristine Li 2 MoO 3 (bond length: 2.02 Å) were split into three different Mo-O bonds (1.68, 2.06 and 2.48 Å) after being charged to Li 0.53 MoO 3 . The Mo–Mo bonds were increased from 2.62 to 2.71 Å, which is not obvious in Fig. 3b , since it overlaps with the longest Mo-O bond. These results further confirmed the distortion of Mo-O 6 octahedral after charge and the expansion along the a and b directions because of the increased Mo–Mo bond length. James and Goodenough [18] revealed that some of Mo ions migrated to the Li layer in Li 2 MoO 3 during delithiation, which is responsible for the formation of the second phase (Phase II). All the three lattice parameters of Phase II are larger than those of Phase I. From the XAS results, we know that the Mo 4+ ions are oxidized to close to Mo 6+ state with a 4 d 0 configuration, which is no longer energetically favourable to stay in the undistorted Mo-O 6 octahedra. They prefer to stay in the distorted Mo-O 6 octahedra [23] or Mo-O 4 tetrahedra [24] . STEM images in Fig. 4a,b provide a clear direct observation of the Mo migration from the transition metal layer to the lithium layer after charge. When a transition metal ion at a 3b site (in the LiM 2 layer) migrates to a 3a site (in the Li layer) in a layered structure, it usually passes through the face-sharing tetrahedral site that connects two edge-sharing octahedra. This movement is easy to occur when the transition metal is at high valence states [13] , since, at such states, its small radius and electronic structure fit well in the intermediate tetrahedral site. On the basis of the in situ XRD, XAS and STEM results, the c parameter breathing of Li 2 MoO 3 during lithium extraction is strongly affected by the migration of Mo ions from 3b sites to 3a sites ( Fig. 4c ). In the Phase I-dominated region, the decreased c/a ratio implies that lithium ions were mainly extracted from the LiMo 2 layer, leading to the solid solution region based on Phase I. After 0.5 Li ions were extracted from Li 2 MoO 3 , Phase II started to grow up and gradually became the dominating phase. This is suggesting that Li ions in Li layers are mainly extracted after most of Li ions in LiMo 2 layers have been extracted. Some of the Mo ions that had been oxidized to close to Mo 6+ state began to move to the neighbouring face-sharing tetrahedral sites. Since electrostatic repulsions would inhibit simultaneous occupancy of face-shared tetrahedral and octahedral sites, a molybdenum ion motion from a 3b octahedral site to a tetrahedral site through a common face can take place only if this tetrahedral site shares faces with three empty octahedral sites. This movement is quite similar to the vanadium ion movement in layered LiVO 2 system during charge [13] . However, for LiVO 2 , the V 5+ ion can only go through the tetrahedral site close to the 3a sites in the Li layer (Path 2 in Fig. 4c ), since all 3b sites are fully occupied by vanadium ions. In the case of Li 2 MoO 3 , since the lithium ions can be extracted from the 3b sites in the LiMo 2 layer, molybdenum ions have the chance to move to the tetrahedral sites nearby 3b sites as well, and then move to the 3a sites (Path 1 in Fig. 4c ), making this type of migration easier. In contrast, this kind of migration does not occur in Li 1− x CoO 2 at room temperature, since tetrahedral site Co 4+ or Co 5+ are not energetically accessible [13] . 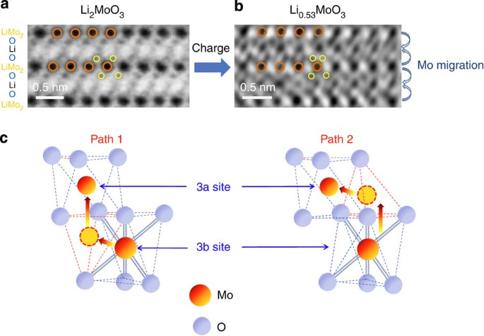Figure 4: Mo migration during the first charge. (a,b) High-resolution annular-bright-field (ABF) STEM images of Li2−xMoO3at pristine (x=0) and fully charged (x=1.47) states, respectively. (c) Two possible Mo ion migration paths from 3b sites to 3a sites in Li2−xMoO3through intermediate tetrahedral sites during charge. Figure 4: Mo migration during the first charge. ( a , b ) High-resolution annular-bright-field (ABF) STEM images of Li 2− x MoO 3 at pristine ( x =0) and fully charged ( x =1.47) states, respectively. ( c ) Two possible Mo ion migration paths from 3b sites to 3a sites in Li 2− x MoO 3 through intermediate tetrahedral sites during charge. Full size image The STEM images in Fig. 4a,b also provide the projection of Mo-O 6 octahedra along the a axis. In pristine Li 2 MoO 3 , Mo-O 6 octahedra are undistorted. After being charged to Li 0.53 MoO 3 , the Mo-O 6 octahedra are highly distorted. On the basis of the XRD and EXAFS results, the schematics of the octahedral distortion before and after charge are shown in Fig. 5a,b . The projection of Mo-O bond expansions are mainly on the a–b plane, which may partially contribute to the increase of a and b parameters. The component of Mo-O bond contractions along the c axis could decrease the lattice parameter c , if only the O–Mo-O slabs are considered. However, similar to the LiCoO 2 system, such contraction is overtaken by the increasing distance of O–Li–O because of the increased repulsion force between the O layers and results in a slightly increased c parameter. The migration of Mo ions from the LiMo 2 layer to the Li layer created ‘cycling-induced cation mixing’. The Mo cations migrated to the Li layer served two important roles in stabilizing the structure during cycling. In the early stage of charging, they fill in the places and play the role of extracted Li ions to ‘glue’ two nearby O layers, reduce the expansion of the c axis; in the late stage at high voltage charging, they serve as ‘pillars’ to prevent the ‘collapse’ of the structure in the c direction. Moreover, Most of Mo cations in the Li layer can reversibly move back to the LiM 2 layer during lithiation process if proper cutoff voltage is applied [25] . 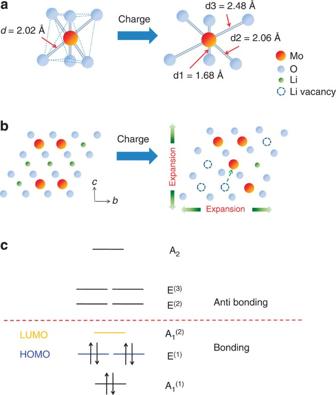Figure 5: Structural evolution of Li2MoO3during the first charge. (a) Schematics of Mo-O6octahedral distortion before and after charge. (b) Schematics of lattice expansion and Mo ion migration during charge. (c) Schematics of molecular orbital levels around the Fermi level and their electron occupation in the Mo3O13cluster. (HOMO is the highest occupied molecular orbital and LUMO is the lowest unoccupied molecular orbital. See more details inSupplementary Fig. 7). Figure 5: Structural evolution of Li 2 MoO 3 during the first charge. ( a ) Schematics of Mo-O 6 octahedral distortion before and after charge. ( b ) Schematics of lattice expansion and Mo ion migration during charge. ( c ) Schematics of molecular orbital levels around the Fermi level and their electron occupation in the Mo 3 O 13 cluster. (HOMO is the highest occupied molecular orbital and LUMO is the lowest unoccupied molecular orbital. See more details in Supplementary Fig. 7 ). Full size image Most of the interpretations of the unit cell breathing of lithium transition metal oxide cathode materials during cycling have been based on the arrangement of ‘hard sphere’ ions with varying radius at different valance states. These interpretations have been successful on most of the ‘normal’ cathode materials such as LiMO 2 , (M=Co, Ni and Mn), LiMn 2 O 4 and LiFePO 4 . However, when the ‘abnormal’ systems, such as Li 2 MoO 3 and LiVO 2 , are considered, this ‘hard sphere’ ion model does not work at all. We believe that electronic structures need to be introduced to explain the behaviour of these ‘abnormal’ materials. Here we present some of our ideas in this new direction and hope to inspire more experimental and theoretical studies. Since Mo 4+ is a 4 d 2 configuration in an octahedral site, two 4 d electrons occupy the low t 2g levels in the octahedral environment. Direct metal–metal bonding has been confirmed between two neighbouring edge-sharing octahedra in the Li 2 MoO 3 system [26] . The strength of metal–metal interactions depends on the cation–cation separation ( R ) and the occupancy of the d orbitals, especially the t 2g set that can be directed towards all the edges of the octahedral coordination polyhedron. Since the direct t 2g − t 2g orbital overlap occurs because of the short Mo–Mo distance (2.62 Å) and diffused 4 d orbitals of the Mo 4+ ion in spherical field, strong metal–metal bonding is formed in Li 2 MoO 3 , evidenced by the Mo 3 triangle clusters with the Mo–Mo bond. The Mo–Mo bond length is even shorter than that in metallic Mo (2.72 Å). When lithium ions were extracted, Mo 4+ was oxidized to higher valence state. The loss of metallic bonding t 2g electrons will weaken the Mo–Mo bond, resulting in longer Mo–Mo bond length. In consequence, the lattice parameters a and b increase during delithiation of Li 2 MoO 3 . In other words, in a system in which metallic bonding is formed, the unit cell breathing will no longer be controlled by the M-O bond length only, but also strongly affected by the M–M bonding change. In case of LiVO 2 and LiNbO 2 , the direct metal–metal bonding was also found in their transition metal slabs [13] , [14] . In addition, according to the molecular orbital theory, the HOMOs (high occupied molecular orbitals) of Mo 3 O 13 clusters in Li 2 MoO 3 are the bonding orbitals [27] ( Fig. 5c and more details in Supplementary Fig. 7 ). Since bonding orbitals bring the atoms close together while antibonding orbitals drive atoms apart, extracting electrons from HOMOs that are bonding in Li 2 MoO 3 would lead to the increase in the Mo–Mo bond length. It should be noted that in LiMO 2 (M=Co, Ni) systems with normal unit cell breathing, HOMOs are the antibonding orbitals. This provides additional supports to the effects of electronic structure on unit cell breathing behaviour from molecular orbit theory point of view. In searching a general rule to categorize the transition metal oxides with ‘normal’ and ‘abnormal’ unit cell breathing, we examined the electronic structures of different transition metal elements contained in these oxides. It was found that in the cathode materials LiMO 2 with ‘normal’ unit cell breathing mode (M=Co and Ni), the transition metal ions usually have more than four electrons in 3 d orbitals (Co 3+ : d 6 ; Ni 3+ : d 7 ). The metal–metal interactions in these systems are very weak because of the localized d orbitals and large M–M distance (usually more than 2.8 Å). The d orbital of two neighbouring metal ions cannot overlap with each other to form the metallic bonding. The unit cell breathing of these systems are dominated by the M-O bonding and the effects of M–M bonding are negligible. During lithium extraction from these systems, the electrons are removed from the antibonding M3 d –O2 p orbital, leading to the shrinking of M-O bond length in MO 6 octahedra and the M–M distance is shortened accordingly. As a result, the a and b lattice parameters in these systems decrease with increasing lithium extraction. Generally, in the periodic table, the diffusion of d orbitals (de-localization) for transition metals decrease with the increasing atomic number in the same period but increase with the increasing atomic number in the same group ( Supplementary Fig. 8 ). The more diffused is the d orbital, the stronger the metal–metal bonding in two edge-sharing MO 6 octahedra ( Fig. 6 ). 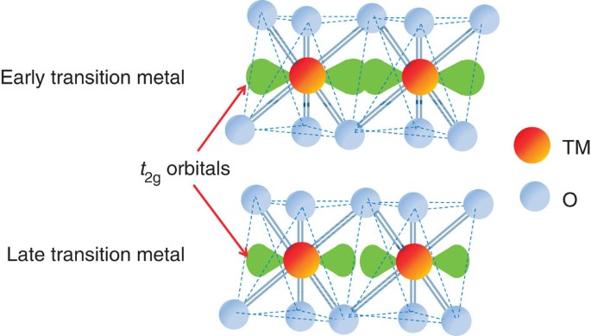Figure 6: Schematics oft2gorbital interactions for transition metals in edge-sharing MO6octahedral. t2gorbital interaction for early transition metals is quite different from that of late transition metals, since thet2gorbital of the later is more localized (TM, transition metal ion; O, oxygen ion.). On the basis of the above the discussion, a rough relationship between the unit cell breathing mode and the electronic structure of transition metals in layered cathode compounds can be proposed as: Figure 6: Schematics of t 2g orbital interactions for transition metals in edge-sharing MO 6 octahedral. t 2g orbital interaction for early transition metals is quite different from that of late transition metals, since the t 2g orbital of the later is more localized (TM, transition metal ion; O, oxygen ion.). Full size image For the late transition metal compounds [28] (VIII groups in the Periodic Table. M x + : d n , n >4), M–O bonds dominates the unit cell breathing mode. They usually show contracted a and b lattice parameters and expanded parameter c during lithium extraction before the collapse of the crystal structure. For the early transition metal compounds [29] (IVB–VIB groups in the periodic table, M x + : d n , n <4), M–M bonding plays more important role on the unit cell breathing mode. They generally show expanded lattice parameters a and b during lithium extraction because of the weakening of the direct metal–metal bonding. The change of parameter c depends on the balance between the expansion of O–Li–O (interslab distance) and the contracting O–M–O length (intraslab distance). In some cases such as Li 2 MoO 3 and LiVO 2 , the significant migration of transition metals to the Li layer also contributes to the evolution of parameter c . For Li 2 MoO 3 , the parameter c expansion in the early stage of charge is much less comparing with those of the late transition metal oxides. For LiVO 2 , the parameter c even reversed normal course into a contraction during charge. This type of transition metal ion migration to the Li layer will also suppress the structure collapse during high voltage charge, providing benefits in both energy density and cycle performance of the cathode, if the potential negative impacts on rate capabilities can be managed. As we all know, the structure degradation of layered cathodes are the main obstacle for developing high energy density LIBs. For today’s state of art commercial cathode materials with layered structures, in order to keep the acceptable capacity retention during cycling, the charge voltage needs to be limited below certain values (normally 4.2 V for LiCoO 2 and 4.3 V for LiNi 1/3 Co 1/3 Mn 1/3 O 2 ). Although charging the cell to a higher voltage limit will be the easiest way to increase the specific energy of the cell, it is not so easy in practice, since it will cause significant capacity fading in subsequent cycles. The main reason of this problem is the excessive unit cell breathing range for the layered structures, especially the collapse of the c parameter during high voltage charging. From this study, we know that the early transition metal compounds have the intrinsic capability to reverse direction or significantly reduce the range of the unit cell breathing during charge–discharge cycling. This unique property can be utilized when certain early transition metals are selected as substituting elements to suppress the unit cell breathing range during cycling. Therefore, by substituting the early transition metal ions in the commercial layered cathode materials (LiCoO 2 , LiNi 1/3 Co 1/3 Mn 1/3 O 2 and so on), it is possible to develop new cathode materials with higher charge voltage limit without significant deterioration of cycling performance. As explained previously, the electronic structures are playing very important roles in determining the unit cell breathing behaviour. As one of the important tools for electronic structure studies, molecular orbit theory provides us more in-depth understanding of the origin and mechanism of such crystal structure changes. In addition, the metal–metal bonding in such systems can also facilitate the electron transportation in the layered structure, having the potential to increase the electronic conductivity [30] . It was also reported that some of the early transition metal ions at high valance states can migrate to Li layers during cycling leading to the formation of a disordered layered structure, which can facilitate the lithium diffusion as some authors proposed in the literature [31] . The transition metal ions that migrated to Li layers can also serve as ‘pillars’ to prevent the collapse of the structure in the c direction during high voltage charging. These results reveal a new strategy to develop high energy density cathode materials for lithium-ion batteries through structural design. They also provide valuable guidance for the research and development of new electrodes for other rechargeable battery systems, such as sodium and magnesium ion batteries. Li 2 MoO 3 synthesis and cell test Li 2 MoO 3 powders were synthesized by reducing commercial Li 2 MoO 4 (Alfa Aesar) at 650 °C for 12 h in flowing H 2 /Ar (10:90 v/v). The detailed synthesis was reported in our recent publications [25] . Cathode specimens were prepared by slurrying the active material with 10 wt % carbon black and 10 wt % poly-vinylidene fluoride in N-methylpyrrolidone solvent, and then coating the mixture on Al foil. After vacuum drying at 60 °C for 24 h, electrode disks were punched and weighed. The cathodes were incorporated into cells with a high-purity lithium metal foil anode and a Celgard separator. LiPF 6 (1 M) in ethylene carbonate and dimethyl carbonate with a volume ratio of 1:1 was used as the electrolyte. The 2,032-type coin cells were assembled in an argon-filled glove box for electrochemical tests. In situ XRD characterization In situ XRD patterns were collected at beamline X14A of the National Synchrotron Light Source (NSLS) at Brookhaven National Laboratory by a linear position sensitive silicon detector. The wavelength used was 0.7747 Å. For in situ XRD experiments, specially designed electrochemical coin cells using kapton film windows on both sides were employed. The two theta angles of all the XRD spectra presented in this paper have been recalculated and converted to corresponding angles for λ =1.54 Å, which is the wavelength of conventional X-ray tube source with Cu-K a radiation, for easy comparison with other published results. In situ XAS characterization and data analysis The in situ Mo K-edge XAS data were collected in transmission mode at beamline X18B at the NSLS and beamline 12BM of Advanced Photon Sources at the Argonne National Laboratory. Energy calibration was carried out using the first inflection point of the reference spectrum of Mo metal foil (Mo K-edge=20,000 eV), which was simultaneously collected during each measurement during the in situ experiments. The XANES and EXAFS spectra were processed using the Athena18 and Artemis19 software packages [32] . The AUTOBK code was used to normalize the absorption coefficient, and to separate the EXAFS signal, χ(k) , from the isolated atom-absorption background. The extracted EXAFS signal, χ(k) , was weighted by k 3 to emphasize the high-energy oscillations and then Fourier-transformed in a k range from 3.5 to 13.5 Å −1 using a hanning window with a window sill ( Δk ) of 1.0 Å −1 , thereby obtaining magnitude plots of the EXAFS spectra in R-space (Å). The Fourier-transformed peaks were not phase-corrected, and thus the actual bond lengths are ~0.3–0.5 Å longer. The filtered Fourier transforms of EXAFS spectra were then fitted using theoretical single scattering paths generated with the FEFF 6.0 ab initio simulation code. TEM characterization The ex situ Cs-corrected STEM measurements of the pristine Li 2 MoO 3 and delithiated Li 2 MoO 3 were conducted on a JEOL 2100F TEM equipped with a CEOS probe aberration corrector (Heidelberg, Germany). The available spatial resolution of the microscope is 90 picometres ( pm at an incident angle of 40 mrad. The raw pictures were treated for noise reduction by ABSF filters. How to cite this article : Zhou, Y.-N. et al. Tuning charge–discharge induced unit cell breathing in layer-structured cathode materials for lithium-ion batteries. Nat. Commun. 5:5381 doi: 10.1038/ncomms6381 (2014).